Impurity-band transport in organic spin valves The central phenomenon in the field of organic spintronics is the large magnetoresistance in thick organic spin valves. A prerequisite for understanding the magnetoresistance is a reliable description of the device resistance, or the I-V characteristics. Here I show that the observed I-V characteristics in the organic spin valves is incompatible with charge injection into the organic’s lowest unoccupied molecular orbital or highest occupied molecular orbital but can be explained by electrons tunnelling into a broad impurity band located in the gap between these molecular orbitals. Voltage drop takes place mainly across depletion layers at the two electrode/organic interfaces, giving rise to electrode-limited charge transport. Spin-dependent electron tunnelling into the impurity band from the ferromagnetic electrodes results in spin accumulations inside the organic, which rapidly diffuses through the organic primarily via the exchange between impurity-band electrons. This picture explains the major magnetoresistance features and predicts enhanced capacitance in these devices. Organic spintronics has attracted considerable interest since the discovery of large magnetoresistance (MR) in thick (~100 nm) organic spin valves (OSVs) [1] , [2] , [3] , [4] , [5] , [6] , [7] . To harness the electron spin in organics for spintronic applications, it is mandatory to elucidate the MR, which in turn requires that the device resistance of the OSVs be adequately accounted for. While the large thickness of the organic film in an OSV precludes a direct tunnelling between the electrodes, the observed I-V characteristic is also incomprehensible in terms of electron injection into the organic’s lowest unoccupied molecular orbital (LUMO) or hole injection into the highest occupied molecular orbital (HOMO), as commonly assumed in literature [1] , [2] , [3] , [4] , [5] , [6] , [7] , [8] , [9] . The two electrodes, labelled 1 and 2, in an OSV have different Schottky barriers, q φ 1 < qφ 2 ( q =| e | is the electron charge), which would give rise to a built-in potential, V bu = φ 2 − φ 1 , in an undoped organic film at zero bias. This structure is essentially a fully depleted Mott diode [10] , [11] , [12] , [13] and, for both electron- and hole-injection devices, charge injection would be more efficient when electrode 1 is the cathode. The current for the electron-injection device under a bias V at temperature T would be [10] Here N C is the density of states, D h the electron hopping diffusion coefficient in the LUMO, L the thickness of the organic film and k B the Boltzmann constant. For a hole-injection device, φ 1 is replaced by E g − φ 2 with E g being the LUMO–HOMO gap of the organic and D h by the hole hopping diffusion constant in the HOMO. The I-V characteristic would be sensitive to the temperature and barrier height, highly nonlinear and asymmetric between positive and negative biases for q | V |/ k B T >1. In particular, at cryogenic temperatures (<20 K) and under low biases (<10 mV), where the observed MR in OSVs is most pronounced [1] , [3] , [5] , [6] , [7] , charge injection, according to equation (1), would be impossible for qφ 1 >0.1 eV. Nor could electrons at the electrodes tunnel into the organic’s LUMO or HOMO, which are far from the electrodes’ Fermi level in energy. Experimentally, however, these OSVs are surprisingly conductive [1] , [5] , [6] , [7] . Furthermore, the measured I-V characteristics is linear and largely symmetric between positive and negative biases up to ±0.1 V ( q | V |/ k B T >50 for T =20 K) or higher, insensitive to the temperature and the organic thickness [1] , [7] , in sharp contrast to the expected behaviour of a Mott diode. To fit the observed symmetric I-V characteristics, the space–charge-limited conduction (SCLC) [14] , j =9 ε ν V 2 /8 L 3 , with ε being the dielectric constant and ν the carrier mobility, is frequently invoked [3] , [15] in the literature. However, the premise of the SCLC is that the supply of carriers from electrodes is unlimited (Ohmic contacts), which seems unlikely from the measured band alignment of OSVs ( qφ 1 , E g − qφ 2 >0.5 eV) [16] . In fact, a large MR should not occur in the SCLC, where, by definition, the (ferromagnetic) electrodes have no effect on transport. Indeed, fitting the MR to the SCLC often yields unjustifiedmagnetization-configuration-dependent mobilities and wildly different mobility values for a same organic material [3] . In addition, the observed little thickness dependence of the device resistance [15] contradicts the strong 1/ L 3 dependence expected from the SCLC. Recent Hanle-effect data in the OSVs [17] further challenge the picture of charge injection into the HOMO or LUMO. The low electron- or hole-polaron mobility in the organic suggests the Hanle effect be seen under a transverse magnetic field as small as B c =10 −6 mT [17] , [18] . However, no Hanle effect is detected up to B =10 mT. The overwhelming inconsistencies enumerated above call for a qualitatively different picture to describe charge and spin transport in the OSVs. Here I propose that in the OSVs carriers are injected into a broad impurity band in the gap between the HOMO and LUMO, and show that the unusual I-V characteristics, the absence of the Hanle effet, and major MR features can be consistently explained by the impurity-band transport. Our work suggests that a careful characterization of these impurities in the OSVs is critical to advance the field of organic spintronics. Model The OSVs with a pronounced MR are usually vertical structures [1] , [2] , [3] , [4] , [5] , [6] , [7] , with the top electrode grown after the deposition of the organic. Lateral ferromagnet–organic-ferromagnet devices, where both electrodes are fabricated before the deposition of the organic, however, are much more resistive and seldom exhibit any spin-valve effect [19] . While the I-V characteristics in the vertical OSVs is drastically different from what is expected from a Mott diode, it is strikingly similar to that of metal–inorganic insulator–metal devices, fabricated in a similar manner as the OSVs. It has been recognized that electrical conduction in these inorganic structures is due not to charge injection into the conduction or valence band of the insulator, but rather, to the extrinsic electrons of the metal atoms or filaments originating from one of the electrodes, that is, the insulator is ‘electroformed’ [20] , [21] . I postulate that the organic in the OSVs is also electroformed, containing high-density impurities. Owing to the disordered nature of the organic, these impurities would form an impurity band with a very broad energy distribution located between the HOMO and LUMO of the organic, as shown in Fig. 1d , which guarantees plenty of states available near the Fermi level of the device even at zero bias. To have a reasonable electron tunnelling current and adequate wave-function overlap for band formation, the distance between adjacent impurities should be within 30 Å, corresponding to an impurity density of 10 19 cm −3 . The impurities might be metal atoms, which serve as donors, or O 2 molecules, which serve as acceptors. The presence of high-density impurities in the OSVs is further supported by the accompanying memory effect [22] caused by charge storage, as in the electroformed inorganic structures [20] , [21] . Such memory effects are not expected from the organic diode of Fig. 1a , where the band does not have a local minimum to keep extra charges inside the organic once a bias is removed. While impurities or deep traps have been shown to influence the MR in the OSVs [23] , the present model suggests that the impurity band due to high-density impurities is responsible for charge/spin transport in the OSVs. 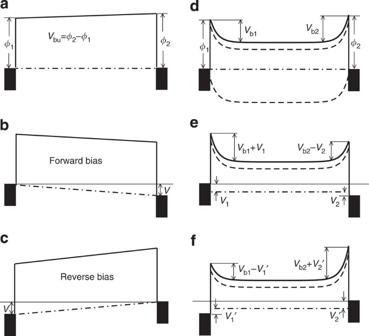Figure 1: Band alignment in an ideal organic structure and in a structure with high-density impurities. The Schottky barriers for the two electrodes areφ1andφ2. From the top to bottom are the band alignment in equilibrium, forward bias and reverse bias, respectively. In the ideal structure, illustrated in (a–c), a built-in potential is developed and the electric field is homogeneous across the device. In the impurity-band structure, illustrated in (d–f), the impurity states are distributed in a broad range between the two dashed lines. Depletion layers form at the electrode/organic interfaces and the corresponding built-in potentials areVb1andVb2. The voltage drops at the two depletion regions areandfor a forward (reverse) bias. Solid and dot-dashed lines describe the LUMO level and the electrochemical potential across the device, respectively. Figure 1: Band alignment in an ideal organic structure and in a structure with high-density impurities. The Schottky barriers for the two electrodes are φ 1 and φ 2 . From the top to bottom are the band alignment in equilibrium, forward bias and reverse bias, respectively. In the ideal structure, illustrated in ( a – c ), a built-in potential is developed and the electric field is homogeneous across the device. In the impurity-band structure, illustrated in ( d – f ), the impurity states are distributed in a broad range between the two dashed lines. Depletion layers form at the electrode/organic interfaces and the corresponding built-in potentials are V b1 and V b2 . The voltage drops at the two depletion regions are and for a forward (reverse) bias. Solid and dot-dashed lines describe the LUMO level and the electrochemical potential across the device, respectively. Full size image Band bending at zero bias Throughout this paper, the OSV structure I consider has two ferromagnets at x <0 and x > L with an organic film sandwiched between them and the electric current is along the x axis. For definiteness I assume that impurities are electron donors. The bending of the impurity band at the metal–organic interface would take place to match the electrode's and the organic’s vacuum levels there, giving rise to built-in potentials V b1 and V b2 near the electrodes. In the interior of the organic, the band bending would be negligible because of the large density of donors, φ 1 − V b1 = φ 2 − V b2 . Such a band diagram was first introduced by Simmons and Verderber [20] to explain the memory effect in the electroformed insulators. The band bending results in formation of depletion layers adjacent to the electrodes with thickness ( i =1,2 and N D is the donor density) and strong electric fields and at the interfaces in equilibrium, as shown in Fig. 1d . To make calculations tractable, the donors are assumed to be uniformly distributed throughout the organic with a fixed value of 10 19 cm −3 . In real devices, the distribution may be quite inhomogeneous with formation of conduction paths or filaments, where the local doping density, that is, the effective N D , can be much higher than the averaged donor density in the organic. Electrical transport under a bias The presence of the impurity band in an OSV indicates that many carriers exist inside the organic at zero temperature before a bias voltage is applied. By contrast none would exist in the ideal organic diode of Fig. 1a . To better understand the charge transport, I temporarily assume that the electrodes in the OSV are nonmagnetic. At cryogen temperatures and under a small forward bias (that is, electrode 1 being the cathode), electrical conduction across the device can be divided into three steps: (1) a net electron flux tunnels from the cathode into the the first layer of impurities adjacent to the cathode, driven by a drop of V 1 in electrochemical potential (ECP); (2) the flux is then conducted by the electrons around the Fermi level within the impurity band inside the organic with an ECP drop of V 3 and (3) the flux tunnels from the last layer of impurities inside the organic into the anode with an ECP drop of V 2 . The total voltage between the anode and the cathode is V = V 1 + V 2 + V 3 . Electron tunnelling currents at steps (1) and (3) can be evaluated by extending the well-known formula [24] , [25] , to the interfacial regions in the OSV. The above equation describes the tunnelling current under a bias of between an electron injector and an electron collector separated by an energy barrier with thickness ℓ and height , measured from the Fermi level of the injector. Here α =4 π (2 m ) 1/2 / h , , m is the electron mass and h is the Planck constant. The electron tunnelling barriers from the two electrodes into the impurity band, as illustrated in Fig. 2 , are determined by the LUMO (conduction-band edge) at a distance of s /2 from the electrodes, where s is the distance between the electrodes and the first impurity layers in the organic. The conduction-band edge, in the vicinity of the two electrodes, can be obtained by noticing that the OSV in Fig. 1d can be viewed as two Schottky diodes in series. Under a forward bias V , the one at the cathode is reverse-biased by V 1 and the one at the anode is forward-biased by V 2 . Their depletion-layer thickness, respectively, increases and decreases, and . The conduction-band edge near the electrodes with respect to their Fermi levels is for 0< x < W 1 and for L − W 2 < x < L . Thus, the barrier heights in steps (1) and (3) are and (note the barrier height in equation (2) is measured from the Fermi level of the injector). 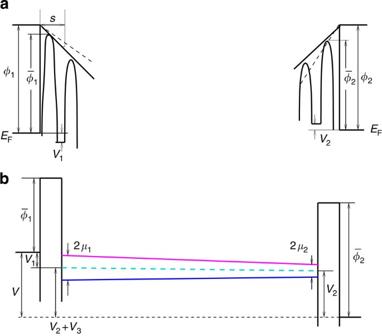Figure 2: Electron tunnelling barriers between the electrodes and their adjacent layers of impurities. Solid and dashed straight lines inadescribe conduction band edge under a bias and in equilibrium. Magenta and blue lines inbare up- and down-spin electrochemical potentials inside the organic, which become degenerate for nonmagnetic electrodes, illustrated by the dashed turquoise line. Consequently, the currents at electrodes 1 and 2 are Figure 2: Electron tunnelling barriers between the electrodes and their adjacent layers of impurities. Solid and dashed straight lines in a describe conduction band edge under a bias and in equilibrium. Magenta and blue lines in b are up- and down-spin electrochemical potentials inside the organic, which become degenerate for nonmagnetic electrodes, illustrated by the dashed turquoise line. Full size image where A 1 ( A 2 ) is the prefactor in equation (2) for electrode 1 (2) multiplying by a geometrical filling factor of the first impurity layers, , with r being the impurity radius. Γ ≃ 2.4 × 10 −3 for N D =10 19 cm −3 and r =1.3 Å. The current in the organic interior can be written as j 3 = V 3 G im = V 3 σ im / L where σ im is the conductivity of the organic because of the impurity-band electrons, which relates to the carrier diffusion constant D im via σ im = q 2 N ( E F ) D im , with N ( E F ) being the density of states at the Fermi level. In the impurity band, electrons use variable-tange hopping with the excitation energy approaching zero near zero temperature [26] , and σ im is finite at zero temperature. For a given voltage V , the three independent unknowns V 1 , V 2 and j can be determined by requiring the three currents be continuous, j 1 = j 2 = j 3 = j . The obtained voltage-drop distribution and I-V characteristics are shown in Fig. 3c,d . I see that the percentage of voltage drop at electrode 1 (2), whose Schottky diode is reversely biased, V 1 / V ( V 2 / V ), increases with the bias for the forward (reverse) bias. The I-V curve is essentially symmetric between forward and reverse biases and linear (see Fig. 4a ). The calculated voltage drop in the organic interior V 3 is negligible as compared with V 1 and V 2 , that is, the charge transport is electrode-limited and is insensitive to the device thickness. The tunnelling transport in equation (2) depends on temperature very weakly. All these features are consistent with the observed I-V characteristics in the OSVs but incompatible with the I-V characteristics expected from an ideal organic diode, as shown in Fig. 3a,b . In particular, the theoretical I-V characteristic is in good agreement with the experimental data of a LaSrMnO/Alq 3 /Co device at T =15 K in ref. 27 . 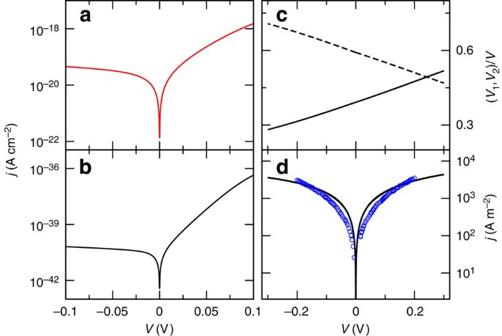Figure 3: I-V characteristics for the Mott diode and for the impurity-band conduction. Panelsa,bcorrespond toT=100 and 200 K for the Mott diode. Panelsc,dare for the impurity-band conduction. Solid and dashed lines incplot the percentage of voltage drop at the electrodes 1 and 2. Black and magenta curves ind, corresponding toT=20 and 300 K, are on top of each other. Circles indare experimental data of an LaSrMnO/Alq3/Co device with the active area of 0.2 mm × 0.2 mm in ref.27. For the Mott diode the parameters areDh=10−5cm2s−1,qφ1=0.8 eV andqφ2=0.9 eV, which mimic a hole-injection LaSrMnO/Alq3/Co device. In the impurity-band model,qφ1=1.6 eV,qφ2=1.7 eV, the barriers for electron injection into the same device. Other parameters areqVb1=0.8 eV,qVb2=0.9 eV,s=1.2 nm,ε=2,ND=1019cm−3,N(EF)=1019cm−3eV−1,L=50 nm,Dim=4.5 × 10−4cm2s−1and Γ=2.4 × 10−3. The electrodes are assumed nonmagnetic. Figure 3: I-V characteristics for the Mott diode and for the impurity-band conduction. Panels a , b correspond to T =100 and 200 K for the Mott diode. Panels c , d are for the impurity-band conduction. Solid and dashed lines in c plot the percentage of voltage drop at the electrodes 1 and 2. Black and magenta curves in d , corresponding to T =20 and 300 K, are on top of each other. Circles in d are experimental data of an LaSrMnO/Alq 3 /Co device with the active area of 0.2 mm × 0.2 mm in ref. 27 . For the Mott diode the parameters are D h =10 −5 cm 2 s −1 , qφ 1 =0.8 eV and qφ 2 =0.9 eV, which mimic a hole-injection LaSrMnO/Alq 3 /Co device. In the impurity-band model, qφ 1 =1.6 eV, qφ 2 =1.7 eV, the barriers for electron injection into the same device. Other parameters are qV b1 =0.8 eV, qV b2 =0.9 eV, s =1.2 nm, ε =2, N D =10 19 cm −3 , N ( E F )=10 19 cm −3 eV −1 , L =50 nm, D im =4.5 × 10 −4 cm 2 s −1 and Γ=2.4 × 10 −3 . The electrodes are assumed nonmagnetic. 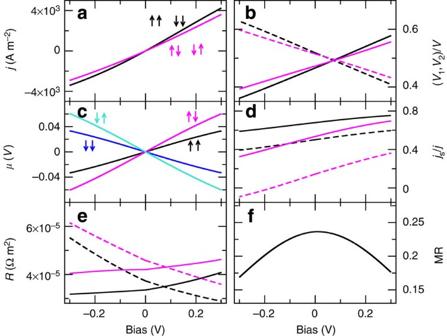Figure 4: Spin and charge transport in an OSV as a function of applied voltage. Panelsa–fdescribe charge current, relative voltage drop, spin splitting in ECP, ratio of spin current and charge current, contact resistance, and MR, respectively. Black and magenta lines correspond to PA and AP configurations, respectively. Solid and dashed lines inb,d,eare for the electrodes 1 and 2, respectively. The spin splittings incat the two electrodes are nearly same. Full size image Figure 4: Spin and charge transport in an OSV as a function of applied voltage. Panels a – f describe charge current, relative voltage drop, spin splitting in ECP, ratio of spin current and charge current, contact resistance, and MR, respectively. Black and magenta lines correspond to PA and AP configurations, respectively. Solid and dashed lines in b , d , e are for the electrodes 1 and 2, respectively. The spin splittings in c at the two electrodes are nearly same. Full size image More insight into charge transport can be gained by expressing the device resistance in terms of those of the two Schottky diodes, R i = V i / j i ( i =1,2), by expanding equations (3) and (4), The opposite signs in front of V 1 and V 2 indicate that with increase in bias, a resistance increase at one Schottky diode is accompanied by a resistance decrease at the other. Consequently, the relative voltage drop at one Schottky diode increases and that at the other decreases with the bias; however, the total resistance is insensitive to the bias, that is, the I-V characteristic is linear over a wide range. The ratio of the total applied voltage to the voltage drop across the reversely biased Schottky diode is (see Methods for derivation) where and . Thus, V / V 1 decreases with a forward bias V , and the coefficient ηξ in front of V is controlled by the Schottky diodes’ characteristics. When the applied bias changes its polarity, the Schottky diode at electrode 2 is reverse-biased. The corresponding ratio V / V 2 has a similar expression as in equation (6), with η replace by η −1 . It should be emphasized that in equation (1) the linear I-V curve region is q | V |< k B T , which is extremely narrow as compared with in the present model. Spin-polarized tunnelling at the electrodes Now I include the magnetizations of the electrodes in an OSV and study spin-dependent transport and the MR. When a spin-polarized current flows into the impurity band in the organic, whose electronic structure is presumably degenerate between up- and downspins, the ECP in the organic becomes spin-dependent because of spin accumulation. In the ferromagnets, because of their very short-spin diffusion lengths, the ECPs can be regarded as spin degenerate [28] . Denoting 2 μ 1(2) as the spin splitting of ECP in the organic at electrode 1 (2), as shown in Fig. 2 , the electron tunnelling barrier for both up- and down-spin electrons injected into the organic from electrode 1, is , whereas the barrier for up- (down-) spin electrons ejected from the organic is , where − V 1 +(−)μ 1 is spin-polarized ECP at the first layer of the impurities. At electrode 2, the barrier for up- (down-) spin electrons injected into the electrode is , and the barrier for both up- and down-spin electrons ejected into the organic is . Thus, the spin-polarized currents at electrodes 1 and 2 are The spin-poarizaed A i ↑(↓) ( i =1,2) originates from the spin-polarized density of states in the ferromagnets and can be used to define the spin polarization at the electrodes, p 1 =( A 1↑ − A 1↓ )/( A 1↑ + A 1↓ ), p 2 =( A 2↑ − A 2↓ )/( A 2↑ + A 2↓ ). The spin-dependent currents in equations (7) and (8) suggest that a spin current is injected into the organic at x =0 − , j s (0 − )= j 1↑ (0 − )− j 1↓ (0 − ) and ejected out of the organic at x = L + , j s ( L + )= j 2↑ ( L + )− j 2↓ ( L + ). The spin splitting of ECP, μ i , is caused by spin injection. When the device is under zero bias, both charge and spin currents are zero, μ i =0, and the OSV is in equilibrium with a common Fermi level throughout the whole device. Spin transport in the organic interior The spin splitting of ECP at the ferromagnet/organic interfaces, μ i , will diffuse into the organic interior according to the well-known spin diffusion equation (28), where L s is the spin diffusion length for the electrons in the impurity band, , with τ s being the spin lifetime and D being the spin diffusion constant. The finite spin lifetime and spin diffusion length are due to spin-orbit couplings [29] or hyperfine interactions [8] , which can also cause magnetic-field effects observed in many nonmagnetic organic devices [30] . In the impurity band, the electron wave functions are localized and there is strong wave-function overlapping between adjacent impurities because of their high density. Consequently, spin motion can use two channels: one is via electron hopping from an occupied state to an unoccupied state, which moves both charge and spin simultaneously and is similar to polaron hopping [8] . The other is via the exchange coupling between occupied electrons, which moves spin but not the charge. The latter dominates over the former when the electron wavefunction overlap between adjacent electron spins is strong, as in the impurity band. Hence, the total spin diffusion constant is D = D ex + D im ≃ D ex (ref. 31 ). For N D =10 19 cm −3 , D ex reaches 1 cm 2 s −1 . The required magnetic field B c to see the Hanle effect is then controlled by D in the impurity band rather than the hopping diffusion constant D h in the LUMO or HOMO. For D =1 cm 2 s −1 , B c ~ Dh /( gμ B L 2 ) ~10–10 2 mT ( g is the electron g-factor and μ B the Bohr magneton) [31] , which explains the absence of the Hanle effect in the OSVs. Since the exchange does not move charge, the dominance of D ex suggests that the electric-field-induced spin drift can be neglected. The general solution to the spin diffusion equation is , where c 1 and c 2 are the unknown coefficients to be fixed by the boundary conditions. The spin splitting in the ECP results in a spin current for 0< x < L , where is the effective spin conductance inside the organic. Since , the effective spin conductance of the organic is high, which can homogenize spin polarization inside the organic efficiently, as shown in Fig. 5 . 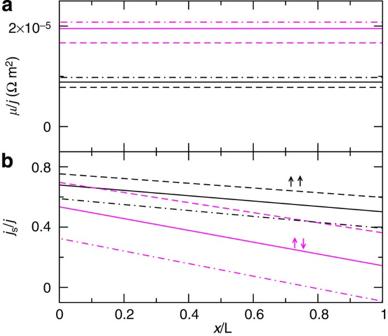Figure 5: Spatial distribution of spin accumulation and spin current in the organic. Panelsa,bplot spin accumulation μ/jand spin-polarization of currentjs/jas a function ofx/L. Black and red lines are for PA and AP configurations, respectively. Solid, dashed and dot-dashed dashed lines correspond toV=0, +0.3 and −0.3 V. The arrow pairs indicate the spin polarizations of the two electrodes.Dex=1 cm2s−1,Ls=2 × 10−3cm,p1=0.8 andp2=0.3. Other parameters are as inFig. 3. Figure 5: Spatial distribution of spin accumulation and spin current in the organic. Panels a , b plot spin accumulation μ/ j and spin-polarization of current j s / j as a function of x / L . Black and red lines are for PA and AP configurations, respectively. Solid, dashed and dot-dashed dashed lines correspond to V =0, +0.3 and −0.3 V. The arrow pairs indicate the spin polarizations of the two electrodes. D ex =1 cm 2 s −1 , L s =2 × 10 −3 cm, p 1 =0.8 and p 2 =0.3. Other parameters are as in Fig. 3 . Full size image Boundary conditions of OSVs In an OSV, the MR is the resistance difference between the parallel (PA) and antiparallel (AP) configurations. In the former, the spin polarizations at the two ferromagnetic electrodes are p 1 and p 2 . In the latter, the spin polarizations are either p 1 and − p 2 or − p 1 and p 2 . To determine the device resistance for the PA and AP configurations, I need to compute the electrical current j under a given applied voltage V . If I neglect any spin relaxation at the interfaces between the organic and the two ferromagnetic electrodes, the spin currents at the interfaces are continuous, j s (0 − )= j s (0 + ) and j s ( L + )= j s ( L − ), where j s (0 − ) and j s ( L + ) are obtained from equations (7) and (8), and j s (0 + ) and j s ( L − ) are obtained from equation (10). In addition, the total electrical current must be constant throughout the device, j = j 1↑ (0 − )+ j 1↓ (0 − )= j 2↑ ( L + )+ j 2↓ ( L + )= V 3 G im . These five conditions completely fix the five unknowns, V 1 , V 2 , c 1 , c 2 and j , for a given bias V . It should be noted that because of spin relaxation in the organic, spin current, unlike charge current, is not continuous throughout the device, as shown in Fig. 5 . Analytical solution near zero bias When the applied voltage approaches zero, equations (7) and (8) can be linearized. If I further neglect the small voltage drop in the organic, V 3 =0, V = V 1 + V 2 , then I can express the device conductance of the PA and AP configurations in a compact form (see Methods for derivation), where , and G 1(2) = G 1(2)↑ + G 1(2)↓ is the effective conductance of the electrodes. . In deriving the equation, we have assumed that ( i =1,2). Accordingly, the MR near zero bias is The above expression illustrates how the spin diffusion length L s enters the expression of MR in an OSV, and shows when , the MR will diminish. Equation (12) provides a theoretical foundation of the widely used empirical formula of MR [1] , [6] , obtained by incorporating spin diffusion in the Julliere formula for tunnelling MR [32] . It further indicates that the MR in an OSV also depends on the effective conductance at the electrodes as well as the effective spin conductance in the organic, which are absent in the empirical formula. This deficiency of the empirical formula frequently manifests itself in the unrealistic p 1 and p 2 values resulted from fitting the MR data to the formula [5] , [15] , [33] . The spin-injection efficiency, that is, the spin polarization of current, at electrode 1 is also found to depend on the conductances of both the electrodes and organic, besides the spin diffusion length in the organic, The expression of the spin polarization of current at electrode 2 can be obtained by swapping indices 1 and 2 in the above equation. Because of spin relaxation inside the organic, j s (0)/ j ≠ j s ( L )/ j . Spin transport under finite biases As the voltage and current increase, more spins accumulate inside the organic, and consequently the spin splittings in the ECPs increase with the voltage, as shown in Figs 4 and 5 . For voltages much smaller than the Schottky barrier heights , the I-V characteristic is linear and spin accumulation increases linearly with V or j . Spins accumulate more in the configuration where spin transport is less efficient, usually in the AP configuration, although opposite situations are also frequently seen in both OSVs and inorganic spin valves (sign anomaly of MR), which has been studied before [34] and is not the focus of this paper. As shown in Figs 4 and 5 , both the spin splittings and spin currents inside the organic depend on the voltage and its polarity. Our model also predicts that the MR decreases with the applied voltage, as shown in Fig. 4f . Since the device resistance is mainly determined by the Schottky diodes at the electrode/organic interfaces, I plot R i = V i / j i ( i =1 and 2) for different biases. I emphasize that this resistance definition remains valid in the presence of spin splitting, which influences the resistance only indirectly by affecting the values of V 1 and V 2 . I see that the resistance R 1 increases with a forward bias and become dominant over R 2 at large biases, but the difference between its values for the PA and AP configurations becomes smaller, while the difference in R 2 changes little. Similarly, for a reverse bias, resistance R 2 becomes dominant at large biases, with its values for the PA and AP configurations becoming closer. This is consistent with experimental measurements, where the MR in most OSVs are found to decrease with the applied bias. The bias dependence of MR can be understood by examining equation (5) for forward bias, where R 1 is dominant in the device resistance. For , I express the MR as (see Methods for derivation) Here ( ) and ( ) are the total current and the spin splitting in ECP at the cathode of the PA (AP) configuration. According to Fig. 4 , and are linear with V , but V / V 1 decreases with V as in equation (6). As a result, the MR approximately follows Δ R / R ≃ 1− γV to the first order of V with γ = ηξ /(1+ η ), that is, decreases with the applied voltage. For reverse biases, the major contribution of the device resistance comes from R 2 , and coefficient γ for the negative bias would become γ ′= η −1 ξ/(1+ η −1 )=ξ/(1+ η ), suggesting a different slope of voltage dependence as compared with the forward-bias case, which explains the asymmetric voltage dependence of MR observed in the OSVs. Thus, our theory relates the voltage dependence of the MR to the device properties and bias directions. In our calculation, only the elastic tunnelling process is included. When inelastic processes involving phonons or magnons become important at elevated temperatures, the MR may decrease more rapidly with the bias. Overwhelming lines of experimental evidence indicate that spin/charge transport in thick OSVs cannot be described as electrons or holes injected into the HOMO or LUMO of the organic. I have proposed an impurity-band model in this paper to describe spin and charge transport in the OSVs. The impurities were unintentionally introduced during the fabrication of the vertical OSVs or by a large bias voltage, and supply plenty of carriers around the Fermi level that facilitate charge and spin transport in the organic. The bottlenecks of electrical transport are at the two electrode/organic interfaces, where electrons tunnel from (into) the electrode into (from) the impurity band of the organic. The impurity band is also present in OSVs fabricated by using ‘soft’ evaporation techniques, as evidenced by the same unusual I-V characteristics observed in those OSVs [27] . This impurity band transport explains the following features of I-V observed in the OSVs. The I-V curves are linear and approximately symmetric for biases up to 0.1 V, and they are insensitive both to the temperature and to the thickness of the organic. By taking into account the spin accumulation inside the organic together with the exchange-induced spin transport, this impurity-band picture explains the following MR features: the MR decays with the thickness of the organic film approximately exponentially and depends on the ratio of contact conductance and the effective spin conductance in the organic; the Hanle effect is suppressed; and the MR decreases with bias and is asymmetric between positive and negative biases. Moreover, the obtained analytic expression of the MR provides a theoretical foundation of the empirical expression used in literature and reveals how the MR and spin-injection efficiency depend on the transport characteristics of organic and electrodes. These results, together with the insight of the anomaly MR sign in the OSVs [34] , constitute an overall understanding of the charge and spin transport in the OSVs. Our model assumes the existence of high-density impurities. These donors/acceptors are too small to be directly seen via transmission electron microscopy and other imaging tools. However, Rutherford backscattering and electron energy loss spectroscopy [35] may help to determine the nature of the donors/acceptors. Another way to detect the impurity band is to measure the device capacitance. The depletion layers near the electrodes suggest that the OSV would have a capacitance of with A being the active area of the device. This capacitance should be much greater than the geometry capacitance C g = εA / L because the depletion layer is ~ W i ~1 nm for N D =10 19 cm −3 , and is much shorter than the orgaic thickness L ~100 nm. Thus, the existence of the high-density impurities and the depletion layers can be verified from AC impedance measurements. In literature, there has been a dispute over whether the carriers in the Alq 3 -based OSVs are electrons and holes [2] , [5] . Alq 3 , the most commonly used organic in the OSVs, is known to be a good electron conductor but an inefficient hole conductor. On the other hand, the HOMO in Alq 3 is usually much closer to the electrode Fermi level than the LUMO, suggesting that hole injection would be more likely. In light of the present model, however, charge injection happens at neither the LUMO nor the HOMO but at the impurity band. Spin-polarized electroluminescence is also reported in an OSV under a large bias, suggesting possible spin organic light-emitting diodes [33] . It should be noted that charge transport under a large bias needed for organic light-emitting diode operation is very different from that under a small bias as in most OSVs. In the former, the strong band bending because of the large bias can enable the SCLC and Fowler–Nordheim field emission, which are unavailable in the latter. The Fowler–Nordheim field emission can drive electrons and holes in the impurity band into the LUMO and HOMO in the organic, giving rise to luminescence. However, since a large percentage of current in the organic is carried by the impurity-band electrons, which do not contribute to luminescence, the quantum efficiency of the luminescence is inherently low. The impurity-band transport picture proposed here suggests the central role of the impurity band in the OSVs. Since the impurity band depends on both impurities and the host organic, spin properties including spin-orbit coupling, hyperfine interaction, spin relaxation and diffusion would be strongly influenced by the nature of impurities. Careful characterization and understanding of these impurities in the OSVs are therefore needed to advance the field of organic spintronics. Numerical approach I numerically solve the nonlinear equations obtained from the boundary conditions of the device model. To ensure stability and accuracy, I gradually ramp up the voltage V and use the solutions for V −Δ V to seek the solutions for V , where Δ V is a small voltage increment. Derivation of equation (6) Since both and V i ( i =1,2) are comparable, the third term is much smaller than the second term and is neglected in equation (6). Analytical solution at small biases When the applied voltage is small, the equations can be linearized, and if I neglect the voltage drop in the organic, V 3 =0, V = V 1 + V 2 , then I can express the spin and charge currents at the interfaces as Using equation (10) in the main text and the boundary conditions, I obtain three linear equations of V 1 , c 1 and c 2 . When the effective conductance is much greater than the conductances G 1 and G 2 , I find the spin splitting in electrochemical potentials are and the device conductance for the PA and AP configurations are obtained from G = j / V , and the MR is The spin-injection efficiencies are the spin polarization of the current Using the approximations, and equations (8) and (9), I obtain the spin-injection efficiency in equation (14). The spin currents at the two electrodes, when , can be expressed as The spatial variation in the spin current is due to the second term. Derivation of equation (15) Expanding the exponential in equation (7) for , I obtain Since the resistance comes mainly from electrode 1, where the Schottky diode is reversely biased, I can estimate the MR from the change the resistance in electrode 1 under a same voltage drop V 1 , How to cite this article: Yu, Z. G. Impurity-band transport in organic spin valves. Nat. Commun. 5:4842 doi: 10.1038/ncomms5842 (2014).